High-resolution three-dimensional partially coherent diffraction imaging The wave properties of light, particularly its coherence, are responsible for interference effects, which can be exploited in powerful imaging applications. Coherent diffractive imaging relies heavily on coherence and has recently experienced rapid growth. Coherent diffractive imaging recovers an object from its diffraction pattern by computational phasing with the potential of wavelength-limited resolution. Diminished coherence results in reconstructions that suffer from artefacts or fail completely. Here we demonstrate ab initio phasing of partially coherent diffraction patterns in three dimensions, while simultaneously determining the coherence properties of the illuminating wavefield. Both the dramatic improvements in image interpretability and the three-dimensional evaluation of the coherence will have broad implications for quantitative imaging of nanostructures and wavefield characterization with X-rays and electrons. As a lensless imaging method, coherent diffractive imaging (CDI) offers great opportunities to image a wide variety of samples [1] , [2] , [3] , [4] in two and three dimensions [5] , [6] with atomic resolution [4] and on ultrafast timescales when used at X-ray free electron laser (XFEL) sources [7] , [8] . CDI works by illuminating a sample with a coherent wavefield after which the coherent diffraction pattern is recorded. The missing phase of the diffracted wave is retrieved through iterative [9] or single-step methods [10] . Paramount to the success of CDI is the use of fully coherent wavefields. Using partially coherent wavefields results in significant unphysical density modulations in the recovered amplitude [2] , [5] , [11] , [12] compromising the verisimilitude of the recovered image. Important applications of CDI include nanoparticle imaging, where quantitative strain mapping can be achieved through the phase of the images [13] . An underlying theme of nanoscience is the emergence of new phases of matter at small sizes [14] and size-dependent phase transitions, which would be detectable as small density variations within the crystals. Strong surface segregation effects expected in alloys would be detected through the density change, as would be surface vacancy proliferation. All of these effects remain unexplored at the present state of development of CDI because the density maps of the images produced are not very reliable. XFEL sources experience shot to shot variations in the coherence properties [15] , potentially limiting their ability for single-shot diffract and destroy imaging. Furthermore, the XFEL pulse transverse coherence lengths are still comparable in size [15] to many objects of interest to CDI, meaning that methods that both characterize the coherence and image simultaneously are needed. Further applications of CDI involve the use of electron sources. These offer the potential for atomic scale imaging [16] of materials, including light elements [17] and biomolecules on ultrafast timescales. However, the coherence lengths of the electron sources are still too small for many samples limiting its potentially enormous applications. Even with the advent of cold sources with improved coherence properties [18] , the lengths are still small compared with many samples of interest. Recently, new research avenues using CDI have been opened by the ability to image both crystalline [19] and non-crystalline [20] samples of arbitrary size in three dimensions using ptychography. The ability to perform these measurements at partially coherent sources (including lab-based X-ray [21] ) or to utilize more flux to reduce the lengthy data acquisition times will be of huge benefit to materials and biological sciences. In addition, the ability to recover the coherence properties of an illuminating beam will find widespread use in characterising optical components [22] for synchrotron or XFEL sources. The CDI method images by inversion of the wavefield diffracted by an isolated object. Isolation of the object ensures that a minimum sampling requirement is met when the diffracted intensity is recorded. If the sample is not sufficiently isolated, the illuminating wavefield can be used to define the extent of the sample [23] while using overlap between adjacent positions that facilitates imaging of extended objects [20] . Essential for CDI is the requirement that the illuminating wavefield is coherent. Many CDI experiments use third-generation synchrotron or electron sources that can be far from fully coherent [24] , [25] . Consequently, there has been recent progress in adapting the current algorithms to accommodate both spatial [26] , [27] and temporal [28] , [29] partial coherence. Until now, these methods have been limited to two dimensions with either complete or partial a priori knowledge of the coherence properties of the illumination. Here, we demonstrate successful inversion of three-dimensional (3D) partially coherent diffraction patterns using a modified iterative algorithm that allows recovery of objects from partially coherent diffraction patterns while simultaneously recovering coherence properties of the illuminating wavefield without a priori assumptions about 3D form. This work identifies an important reason for the failure of current methods and demonstrates a way to obtain dramatic improvements in the presence of less-than-ideal coherence. The method described here is applicable to all applications of iterative CDI, including those from synchrotron, XFEL or electron sources covering 2D and 3D imaging including ptychography. Partial coherence Under the far-field approximation, the diffracted intensity, I ( q ), from a sample's complex electron density, ρ ( r ), for spatially coherent monochromatic plane wave radiation is given by where r is a sample space coordinate, q is a reciprocal space coordinate, is the complex scalar diffracted wavefield given by, . Iterative algorithms are used to recover the phase of by enforcing constraints in the detector and sample plane. The first of the two more common constraints is the modulus constraint, which requires that the amplitude of the wavefield at the detector agrees with that measured (from its intensity). The second constraint is the support constraint, which assumes a priori that the sample is finite in extent. When the radiation is partially coherent, the diffracted intensity is now given by [24] where J ( r 1 , r 2 ) is the mutual optical intensity (MOI), γ || embodies the temporal (or longitudinal) coherence properties relating to the monochromaticity of the wavefield and || indicates the direction parallel to the wavefield propagation. The MOI described by the generalized Schell model [30] is given by, where ψ i is the illuminating wavefield and γ ┴ captures the coherence properties transverse (┴) to the direction of wavefield propagation. The function γ=γ ┴ γ || is the normalized mutual coherence function (MCF), which under the limit of full coherence is equal to unity everywhere. We note that the generality of equation 4 allows both planar and curved wavefronts, such as those found in Fresnel CDI [31] . The recorded partially coherent intensity is now given as a convolution [11] , [24] , where I c ( q ) is the coherent intensity and is the Fourier transform of the normalized MCF. For the case of a dynamic γ , as could be found from recording many shots from an identical sample with an XFEL, equation 5 would become, where ‹ I pc ( q )› is the accumulated intensity and is the 'average' of the MCF at the detector (see Supplementary Methods for derivation). The effect of equation 5 is to blur the coherent intensity by convolving it with the Fourier transform of the normalized MCF [11] , [24] . The partially coherent diffraction pattern is no longer the modulus of the diffracted wavefield, which results in there being no object that will simultaneously satisfy the modulus and support constraints [24] , [32] . Depending on the degree of degradation, the iterative algorithms can produce reconstructions that contain artefacts, non-unique solutions or fail to converge at all [5] , [11] , [26] , [29] , [32] . It is for these reasons that methods that can recover objects from their partially coherent diffraction patterns in three dimensions without a priori assumptions about 3D form are required. Description of experiment To demonstrate simultaneous recovery of a sample and the normalized MCF of the illumination from 3D diffraction data, an experiment was carried out at beamline 34-ID-C at the Advanced Photon Source in Chicago (for further details, see Methods). The sample consisted of Au nanocrystals several hundred nanometres in diameter. Slits in the beamline were used to adjust the MCF. Data were recorded at two different slit settings, 12.5 and 50 μm, chosen to achieve the horizontally 'coherent' and 'partially coherent' illumination conditions, respectively. 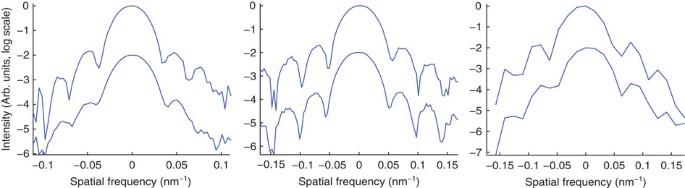Figure 1: Gold nanocrystal diffraction pattern lineouts. Line-outs through the centre of the diffraction pattern of a gold nanocrystal measured under two coherence conditions. The 'high coherence' (top line) and 'low coherence' (bottom line) data are displayed on the same plot. From left to right,Ipc(q1,0,0),Ipc(0,q2,0) andIpc(0,0,q3). The lower line-out has been offset for clarity. Figure 1 shows line-outs taken through the 3D recorded intensity. Degradation in fringe visibility is clearly visible in the horizontal detector direction ( q 1 ), which in the geometry for this experiment is most affected by a change in horizontal coherence. Shown in Supplementary Fig. S1 is a comparison of the reconstructed data to that measured for the low-coherence data set. Figure 1: Gold nanocrystal diffraction pattern lineouts. Line-outs through the centre of the diffraction pattern of a gold nanocrystal measured under two coherence conditions. The 'high coherence' (top line) and 'low coherence' (bottom line) data are displayed on the same plot. From left to right, I pc ( q 1 ,0,0), I pc (0, q 2 ,0) and I pc (0,0, q 3 ). The lower line-out has been offset for clarity. Full size image Reconstruction procedure In order to accommodate partial coherence the modulus constraint needs to be modified. Modification of the modulus constraint has proven successful in accommodating partial temporal [28] , [29] and spatial [26] coherence using modal techniques. The modal methods assume that the recorded diffraction is made up of a number of modes, with the estimate at the recorded diffraction being the incoherent sum of each mode's intensity. Other modifications of the modulus constraint have successfully been incorporated for dynamic sample imaging [33] and molecular damage from XFELs [34] . Ten reconstructions were carried out for each of the slit settings, each starting with a random phase for the wavefield at the detector. All reconstructions used the same recipe which consisted of 10 iterations of error reduction [9] , then 160 iterations of hybrid input–output [9] using β =0.9, and then 40 iterations of error reduction. The support was updated every fifth iteration using shrink wrap [35] . For each of the random starts, two reconstructions were carried out; the first used the usual modulus constraint and the second used the modified modulus constraint given by equation 7 and equation 8. was updated every 15 iterations using the iterative Richardson–Lucy (RL) algorithm (Methods). The reconstructions (including determination of the MCF) were performed in reciprocal space coordinate system after which each reconstruction was transformed to an orthogonal laboratory reference frame with x,y directions being transverse to the beam direction z ( Supplementary Methods ). 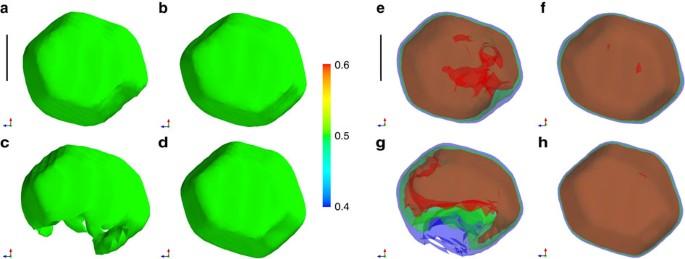Figure 2: Isosurfaces of the reconstructed nanocrystal for differing coherence conditions. (a–d) Opaque isosurfaces (50% of the maximum) of the reconstructed nanocrystal for differing coherence conditions. (a) Imaged under high-coherence conditions assuming full coherence and (b) using the partially coherent modulus constraint. Images from the low-coherence conditions assuming full coherence (c) and using the partially coherent modulus constraint (d). (e–h) Transparent isosurfaces (40–60% of the maximum) of the reconstructed nanocrystal for differing coherence conditions. (e) Imaged under high-coherence conditions assuming full coherence and (f) using the partially coherent modulus constraint. Images from the low-coherence conditions assuming full coherence (g) and using the partially coherent modulus constraint (h). The viewing plane isz–x(blue and red arrows, respectively) and the black scale bar represents 100 nm. 3D reconstructions of gold nanocrystals Figure 2a–d shows a typical reconstructed image of the gold nanocrystal comparing the amplitude (shown as an isosurface at 50% of the maximum) for the high- (a and b) and low-coherence (c and d) data sets assuming perfect coherence (a and c) and accommodating partial coherence (b and d). It is quite clear that, without correcting for the partial coherence, the reconstructed image suffers from significant unphysical density modulations, manifesting itself as a missing segment at the contour level shown (c). On the other hand, the reconstruction accommodating the partial coherence (d) represents the expected shape for a defect-free nanocrystal of uniform density. This is also in agreement with the high-coherence reconstruction (a and b). Also shown in Fig. 2e–h are transparent isosurfaces of the recovered amplitude. The clearly observable variations in density have been reported before [2] , [5] , [11] , [12] with the high-density regions being labelled as 'hot spots'. The hot spots were attributed to partial coherence effects owing to beamline window placement [11] . The coherence-corrected images (f and h) show a much more uniform interior with a well-faceted crystal shape compared with those assuming full coherence (e and g). Shown in Fig. 3 are histograms of the reconstructed amplitude for points within the crystal. The low-coherence histogram (c) has a significantly broader distribution of values compared with the high-coherence (a) and corrected cases (b and d). A Gaussian was fitted to the histogram of the amplitude values. The standard deviation (s.d.) of the distribution improved by a factor of 2.7 and 3.9 for the high- and low-coherence reconstructions, respectively, after using the partially coherent modulus constraint. The phase of the reconstructed nanocrystal is almost unaffected, presumably because it is quite slow-varying. Shown in Supplementary Fig. S2 is the error metric, which quantifies the difference between the reconstructed estimate for the data and that measured. We see a reduction in the error metric of 14% using the partially coherent reconstruction method compared with assuming full coherence. Importantly, these results also show us that significant improvements can be made even to the high-coherence data by incorporating a partially coherent modulus constraint. We attribute this to the fact that the longitudinal coherence was the same for both data sets. The resolution in each direction of the final images was estimated by fitting a Gaussian function to the derivative of the edge of the reconstructed nanocrystal. The resolution (2 σ ) was 17, 8 and 14 nm for x , y and z directions, respectively. A second nanocrystal was also studied using a horizontally partially coherent illumination and found to show the same improvement. Figure 4 shows a comparison between the reconstructions assuming full coherence and accommodating the partial coherence, demonstrating a marked improvement when accommodating the partial coherence using the method outlined here. 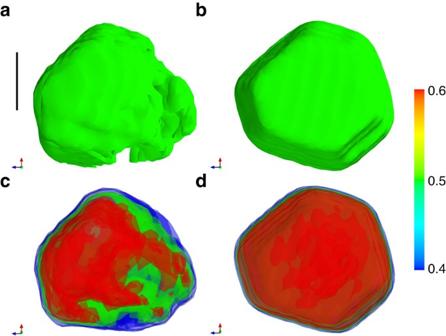Figure 4: Isosurfaces of a second reconstructed nanocrystal taken with partially coherent illumination. (a) Shown is an opaque isosurface (50% of the maximum) assuming full coherence, which is compared with the reconstruction using the partially coherent modulus constraint shown in (b). Transparent isosurfaces (40–60% of the maximum) of the second reconstructed nanocrystal assuming full coherence (c) and using the partially coherent modulus constraint (d). The viewing plane isz–x(blue and red arrows, respectively) and the black scale bar represents 100 nm. The improvements are found to be fully 3D, as can be seen in Supplementary Movie 1 and Supplementary Movie 2 , which show the reconstruction assuming full coherence and accommodating the partial coherence, respectively. Figure 2: Isosurfaces of the reconstructed nanocrystal for differing coherence conditions. ( a – d ) Opaque isosurfaces (50% of the maximum) of the reconstructed nanocrystal for differing coherence conditions. ( a ) Imaged under high-coherence conditions assuming full coherence and ( b ) using the partially coherent modulus constraint. Images from the low-coherence conditions assuming full coherence ( c ) and using the partially coherent modulus constraint ( d ). ( e – h ) Transparent isosurfaces (40–60% of the maximum) of the reconstructed nanocrystal for differing coherence conditions. ( e ) Imaged under high-coherence conditions assuming full coherence and ( f ) using the partially coherent modulus constraint. Images from the low-coherence conditions assuming full coherence ( g ) and using the partially coherent modulus constraint ( h ). 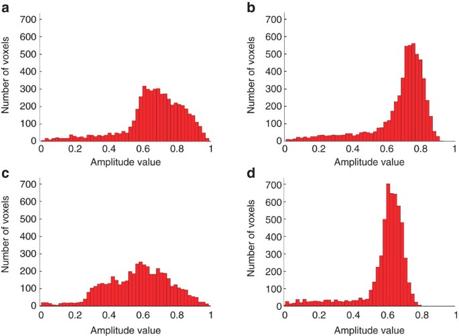The viewing plane is z – x (blue and red arrows, respectively) and the black scale bar represents 100 nm. Figure 3: Histograms of amplitude values of pixels within the crystal. The high-coherence conditions assuming full coherence (a) and using the partially coherent modulus constraint (b). The histograms for the low-coherence reconstructions assuming full coherence (c) and using the partially coherent modulus constraint (d). Full size image Figure 3: Histograms of amplitude values of pixels within the crystal. The high-coherence conditions assuming full coherence ( a ) and using the partially coherent modulus constraint ( b ). The histograms for the low-coherence reconstructions assuming full coherence ( c ) and using the partially coherent modulus constraint ( d ). Full size image Figure 4: Isosurfaces of a second reconstructed nanocrystal taken with partially coherent illumination. ( a ) Shown is an opaque isosurface (50% of the maximum) assuming full coherence, which is compared with the reconstruction using the partially coherent modulus constraint shown in ( b ). Transparent isosurfaces (40–60% of the maximum) of the second reconstructed nanocrystal assuming full coherence ( c ) and using the partially coherent modulus constraint ( d ). The viewing plane is z–x (blue and red arrows, respectively) and the black scale bar represents 100 nm. Full size image The full 3D normalized MCF is also recovered. Line-outs, averaged from 10 random starts, for the horizontal ( x ) and longitudinal ( z ) normalized MCF are shown in Fig. 5 along with a 2D x – z slice for the low-coherence data set. The horizontal coherence length, which can be read off as a characteristic width of these distributions, is 220 nm (defined as the half-width at half maximum (HWHM) of |γ|). This compares well with the value range of 200–300 nm estimated from the beamline geometry ( Supplementary Methods ). The recovered longitudinal HWHM is 485 nm (extrapolated from fitting a Guassian), which compares well with a previously measured [12] HWHM of 660 nm for the same beamline. It is also seen that the HWHM of the horizontal coherence function increases by ~60% from the low- (blue line) to the high-coherence (red line) data set ( Fig. 5a ). There is excellent agreement between the recovered longitudinal normalized MCF from the low- (red line) and high-coherence (blue line) data sets ( Fig. 5b ). We note that no a priori form or model was assumed in this analysis. The source size and beamline optics will largely predict the coherence properties of the illumination. Our result shows that we can obtain an estimate of the coherence properties of the wavefield while simultaneously reconstructing an image of the sample. 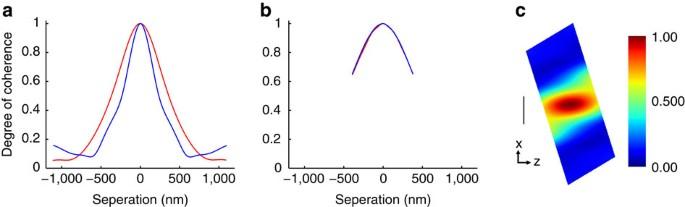Figure 5: Line-outs through the centre of the recovered coherence function in the plane of the sample. Shown is the recovered coherence function for thex(a) andz(b) directions for the high- (red line) and low-coherence (blue) data sets. Also shown (c) is anz–xslice through the recovered coherence function for the low-coherence data set. The black scale bar represents 500 nm. Figure 5: Line-outs through the centre of the recovered coherence function in the plane of the sample. Shown is the recovered coherence function for the x ( a ) and z ( b ) directions for the high- (red line) and low-coherence (blue) data sets. Also shown ( c ) is an z–x slice through the recovered coherence function for the low-coherence data set. The black scale bar represents 500 nm. Full size image Our coherence-correcting method, demonstrated here, has broad implications for CDI as it allows objects to be reconstructed to high resolution in three dimensions when their diffraction patterns have been recorded under less than ideal spatial and/or temporal coherence. This will enable a wider range of samples from all areas of science, including both materials and biological samples, to be imaged as previous limitations on the coherence of the source have been significantly reduced. The method is simple and intuitive, and it is anticipated that it will be adopted widely in the many guises of CDI including high-resolution imaging using synchrotron, XFEL, electron and lab-based X-ray sources of isolated and extended objects (using ptychography) in two and three dimensions. Our coherence-correcting method has the additional benefit of recovering the full 3D coherence properties of the illumination without the need for a priori information. Because of the non-orthogonal coordinate transformation in the Bragg geometry, of which full details are provided in the Supplementary Methods , the transverse and longitudinal directions of the coherence do not align with the simple viewing directions, so a full determination of these requires a full 3D deconvolution. Wavefront propagation methods are seriously compromised by the effects of partial coherence. Knowledge of the full 3D coherence properties of a beam is therefore particularly useful for the characterization of wavefields. This methodology can then be used to assess the quality of beamline optics for synchrotron and XFEL sources. We note this has not been achieved by any other method before to this level of detail. Sample preparation To make the nanocrystals, a 2 nm layer of Ti was deposited using thermal evaporation onto an Si wafer followed by 20 nm of Au. The thin film was then annealed in air at 1,000 °C for ~10 h after which time the film had dewetted and formed nanocrystals. Experiment The sample was placed on a diffractometer and illuminated by 8.9 keV X-rays. To record the diffraction from the nanocrystals, a 1350×1300 pixel charge-coupled device with 20 μm 2 pixels was placed 550 mm from the crystal centred about one of the (111) Bragg peaks. A set of Kirkpatrick–Baez mirrors with focal lengths of 100 and 200 mm in the horizontal and vertical directions, respectively, were used to focus the illumination onto the sample. Approximately 600 mm in front of the sample, roller blade slits were used to aperture the X-ray wavefield in the horizontal direction. Opening and closing the roller blade slits allowed adjustment of the MOI incident on the Kirkpatrick–Baez mirrors. To record the 3D diffraction pattern, the nanocrystals were rocked in 50 0.02° steps with each frame exposed for a total of 16 seconds. Phase retrieval algorithm In order to accommodate partial coherence and simultaneously determine the coherence function, the following algorithm was employed. At iteration k , propagate ψ k ( r ) to the detector plane to obtain . Update the estimate of and then form the current estimate of the measured partially coherent data using: where . Apply the modulus constraint to , using the measured data I pc ( q ) via: After the modus constraint, is propagated to the sample plane. Once in the sample plane real space constraints are enforced, forming the next iterate. The above steps constitutes a single iteration, with the algorithm being run for a prescribed number of iterations. The iterative RL algorithm [36] , [37] was employed to update a numerical estimate of using the measured intensity, I pc ( q ), and a combination of the current and previous iterates estimate of the coherent intensity, . The iterative scheme for is given by, where i is the sub iteration number relating to the coherence function determination. In the limit of full coherence, γ → δ (where δ is the Dirac delta function) and equation 8 becomes the usual modulus constraint that sets the amplitude of the iterate to square root of the measured intensity while retaining the phase. The coherence function was updated every 15 iterations with the RL algorithm run for 25 iterations per update. Increasing the number of iterations had minimal effect on the final result. Twenty-five was found to be adequate to converge to a solution while reducing computation time. The unambiguous separation of a reconstructed object and a MCF, as we demonstrate here, may appear to be an over interpretation of a single set of measurements. We note that the Fourier transform of the object and the MCF affect different general features of the diffraction pattern: the former determines the fringe spacings and their relative positions, while the latter affects their visibility or contrast. As with all deconvolution problems, it is expected that there will be a limited range of applicability of our method to the level of partial coherence that can be corrected. This limit has not been fully established but is likely to be when the normalized MCF reaches zero across , indicating that the normalized MCF must be non-zero across a width twice the size of the object. Furthermore, we note that a relatively tight (reciprocal space) point-spread function has vastly fewer degrees of freedom than the full diffraction pattern. By using the RL algorithm, which seeks a solution that maximizes the entropy rather than a least squares solution, we avoid the situation where when which would occur if , where is the Fourier transform operator. This situation is further avoided by determining from an intensity that is not equivalent to I k unless the solution has been reached. This can be seen that unless . This method is generally robust to noise as the majority of the power in the diffraction patterns are contained within the first few diffraction peaks, where the signal to noise ratio is highest. How to cite this article: Clark, J.N. et al . High-resolution three-dimensional partially coherent diffraction imaging. Nat. Commun. 3:993 doi: 10.1038/ncomms1994 (2012).